Measurement of the first ionization potential of astatine by laser ionization spectroscopy The radioactive element astatine exists only in trace amounts in nature. Its properties can therefore only be explored by study of the minute quantities of artificially produced isotopes or by performing theoretical calculations. One of the most important properties influencing the chemical behaviour is the energy required to remove one electron from the valence shell, referred to as the ionization potential. Here we use laser spectroscopy to probe the optical spectrum of astatine near the ionization threshold. The observed series of Rydberg states enabled the first determination of the ionization potential of the astatine atom, 9.31751(8) eV. New ab initio calculations are performed to support the experimental result. The measured value serves as a benchmark for quantum chemistry calculations of the properties of astatine as well as for the theoretical prediction of the ionization potential of superheavy element 117, the heaviest homologue of astatine. Astatine (At) is the rarest naturally occurring element on earth with an estimated total abundance of 0.07 g (refs. 1 ). There is significant interest in the pharmaceutical use of the isotope 211 At because its decay properties make it an ideal short-range radiation source for targeted alpha therapy in cancer treatment [2] , [3] , [4] , [5] . As only ultra-trace quantities can be used for experimental chemical studies, computational chemistry is an invaluable resource for improving our understanding of At chemistry [6] , [7] . Such computations benefit greatly from validation provided by experimental measurements, as summarized in Brown [8] and Nefedov et al . [9] One of the most important properties is the binding energy of the outermost valence electron which determines the chemical reactivity of an element and, indirectly, the stability of its chemical bonds in compounds. This energy is also referred to as the first ionization potential (IP). Of all the naturally occurring elements, At is the only one whose IP has not been experimentally deduced. However, the IP(At) had been calculated through the use of various theoretical treatments [10] , [11] , [12] , [13] , [14] , [15] . 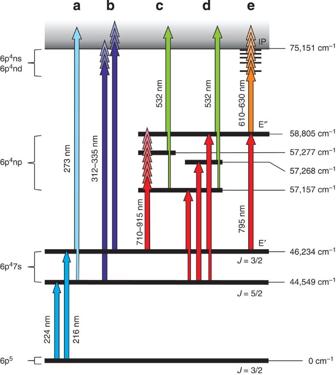Figure 1: Schematic overview of the investigated ionization paths. The assignments of the three lowest levels is according to17. (a) Verification of the two transitions from the ground state atλ1=216 and 224 nm. (b) Ionization threshold: scan of the ionizing laser wavelengthλ2. (c) Development of a three-colour scheme: scan ofλ2in the infra-red region for second excited states starting withλ1=216 nm first step. (d) Verification of the levels found by exciting via theλ1=224 nm first step. (e) Rydberg series: a wavelength scan of the ionizing laser (λ3) in the visible range using the {216; 795;λ3} excitation path. Early extrapolations from the IP data for neighbouring elements gave values of IP(At) from 9.2 to 10.4 eV [10] , [11] , [12] , [13] , however, recent, more precise theoretical treatments [14] , [15] cluster around 9.3 eV ( Table 1 ). Regarding the prediction of IPs of heavier elements and in particular the superheavy elements, the inclusion of relativistic and correlation effects are of major importance. A measurement of the IP for At, the nearest lighter homologue of the recently discovered element with Z =117 (refs. 16 ), therefore provides an experimental basis for developing theoretical methods which incorporate these effects. Table 1 Calculated and experimental values (last two rows) for the first IP of astatine. Full size table The most precise method for determining IPs is the analysis of the converging series of atomic energy levels with a high principal quantum number n , known as Rydberg states. The Rydberg series of an atom can be observed most easily in the ionization spectrum of the final transition of a step-wise resonant ionization scheme. Before this work, the only available data on the optical spectrum of At came from absorption spectroscopy of a 70 ng sample of the artificially produced, longest living (up to 8.1 h) isotopes 209–211 At. Two optical lines at 216.225 and 224.401 nm were observed [17] . This rudimentary knowledge of the atomic spectrum and the lack of a suitable spectroscopic setup in proximity of an isotope production facility limited the feasibility of a measurement of the IP of At. In this article, we report on in-source laser resonance ionization spectroscopy studies of At isotopes using the resonance ionization laser ion source (RILIS) [18] , [19] of the ISOLDE radioactive ion beam facility [20] at CERN. As an initial step, the first experimental value of the IP of the At atom is derived from a direct measurement of the photoionization threshold. This result facilitates the search for additional atomic transitions during the development of an efficient three-colour resonance laser ionization scheme, necessary for the production of pure and intense At + ion beams at ISOLDE. The use of a suitable second-step atomic transition enables resonance ionization spectroscopy of high-lying Rydberg states, resulting in a more precise determination of the IP(At). The extracted value serves as an important benchmark for ab initio calculations in atomic physics and quantum chemistry. New calculations of the IP of At are performed in this work which compare well with the experimental value. First step transitions The tentative assignments of the two spectral lines at λ 1 =216 and 224 nm to transitions from the At atomic ground state, as reported in McLaughlin [17] , were confirmed by resonance ionization laser spectroscopy in a two-colour laser scheme denoted as { λ 1 ; 273}, cf. Fig. 1a . Figure 1: Schematic overview of the investigated ionization paths. The assignments of the three lowest levels is according to [17] . ( a ) Verification of the two transitions from the ground state at λ 1 =216 and 224 nm. ( b ) Ionization threshold: scan of the ionizing laser wavelength λ 2 . ( c ) Development of a three-colour scheme: scan of λ 2 in the infra-red region for second excited states starting with λ 1 =216 nm first step. ( d ) Verification of the levels found by exciting via the λ 1 =224 nm first step. ( e ) Rydberg series: a wavelength scan of the ionizing laser ( λ 3 ) in the visible range using the {216; 795; λ 3 } excitation path. Full size image Figures 2a show laser scans across both of the two first step transitions. The photo-ion rate of 199 At, obtained from α-decay rates, measured by the silicon detector of the Windmill system (see Methods section), was recorded for successive laser scanning steps of λ 1 while λ 2 was fixed at 273 nm, chosen such that the total photon energy is higher than most of the theoretical expectations of the IP of At (cf. Table 1 ). 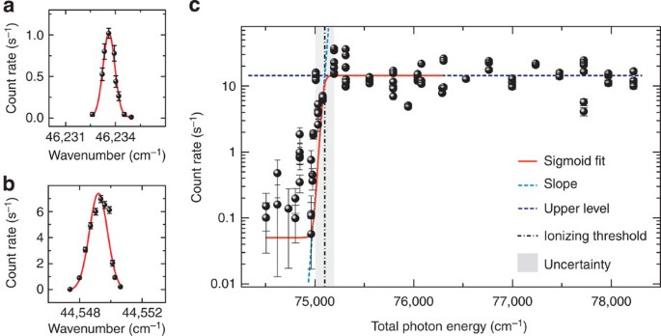Figure 2: Laser scans for the two-step ionization scheme. Panelsaandbshow laser scans across the two optical transitions atλ1=216 andλ1=224 nm, obtained using the ionization path shown inFig. 1aand α-decay detection of the photo-ionized199At. (c) Measurement of the ionization threshold. The count rate of α-particles from the decay of199At is registered for different total photon energies of the applied laser beams used in the two-colour schemes {216;λ2} and {224;λ2} (cf.Fig. 1b). Figure 2: Laser scans for the two-step ionization scheme. Panels a and b show laser scans across the two optical transitions at λ 1 =216 and λ 1 =224 nm, obtained using the ionization path shown in Fig. 1a and α-decay detection of the photo-ionized 199 At. ( c ) Measurement of the ionization threshold. The count rate of α-particles from the decay of 199 At is registered for different total photon energies of the applied laser beams used in the two-colour schemes {216; λ 2 } and {224; λ 2 } (cf. Fig. 1b ). Full size image Ionization threshold The two-colour ionization schemes {216; λ 2 } and {224; λ 2 }, as illustrated in Fig. 1b , were applied for scanning the second-step laser wavelength within the range λ 2 =312–335 nm, which encompasses the most recent published theoretical predictions of the IP including the value from Chang et al . [15] , privately communicated before publication. Figure 2c reveals the onset of photoionization at a total excitation energy of around 75,000 cm −1 . The position of the photoionization threshold, denoted as the vertical dotted line, was determined as the intersection of the slope (blue tilted line) at the inflection point of a fitted sigmoid curve (red line) and its upper level (blue horizontal line). Using this method we obtain IP thr. (At)=75,129(95) cm −1 , corresponding to 9.315(12) eV. The quoted uncertainty arises from the low statistics. Three-colour ionization scheme The development of a three-colour ionization scheme, which required a search for intermediate atomic transitions, resulted in an increased ionization efficiency and enabled high-resolution laser scans across the ionization threshold. The search for new second-step transitions ( λ 2 ) to higher lying atomic states, was performed at the TRIUMF-ISAC radioactive ion beam facility with the TRILIS laser ion source [21] . The fundamental output of a widely tunable grating-based Ti:sapphire (Ti:Sa) laser [22] was used to scan λ 2 between 710 and 915 nm in a three-colour scheme {216; λ 2 ; 532}, see Fig. 1c . Three new transitions were discovered. These transitions were subsequently confirmed at ISOLDE where ionization routes via both the λ 1 =224 nm and λ 1 =216 nm first steps were studied by laser spectroscopy of the 205,196 At isotopes. In total six new transitions between excited states of At have been observed. An overview is given in Fig. 1c , further details of these will be published elsewhere. Spectroscopy of Rydberg states The {216; 795; λ 3 } excitation path was used for the scan of the third step ( λ 3 ) across the ionization threshold, as given in Fig. 1e . For this study, the ISOLDE RILIS Ti:Sa laser system was arranged to produce the two laser beams necessary to populate the E ′′ level (cf. Fig. 1 ). The transition energies of the intermediate states are ν ′=46,234.0(3) cm −1 and ν ′′=12,571.5(3) cm −1 , obtained from Gaussian fits of several laser scans across the 216 and 795 nm resonances of 205 At. From these we obtain E ′′= ν ′+ ν ′′=58,805.4(5) cm −1 . A synchronized dye laser provided the third step laser radiation and was set to a tuning range encompassing the previously localized region of the ionization threshold. The dye laser was scanned whilst the 205 At ion current was directly measured with a Faraday cup (FC). A series of more than 30 Rydberg levels was observed in the λ 3 scan range of 15,000–16,300 cm −1 , as shown in Fig. 3a . 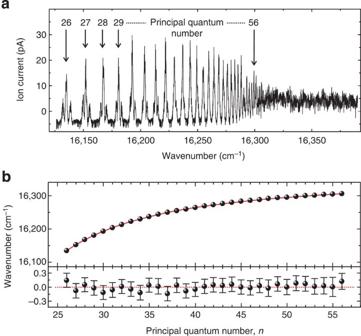Figure 3: Determination of the ionization limit of the excited state. (a) Laser scan of the ionizing laser across the ionization threshold of At. The observed Rydberg resonances converge towards the ionization limit. The indicated principal quantum numbers (n) are based on the assumption of anndseries. (b) Analysis of the observed Rydberg spectrum. The top panel shows the position of 31 high-lying Rydberg levels. The Rydberg formula is fitted to the positions of the main peaks in the multiplets belonging to differentn. The residuals of the fit are shown in the bottom panel. Figure 3: Determination of the ionization limit of the excited state. ( a ) Laser scan of the ionizing laser across the ionization threshold of At. The observed Rydberg resonances converge towards the ionization limit. The indicated principal quantum numbers ( n ) are based on the assumption of an nd series. ( b ) Analysis of the observed Rydberg spectrum. The top panel shows the position of 31 high-lying Rydberg levels. The Rydberg formula is fitted to the positions of the main peaks in the multiplets belonging to different n . The residuals of the fit are shown in the bottom panel. Full size image The Rydberg atoms were ionized inside the hot cavity ion source by the residual laser light, black-body radiation or by collision processes. The Rydberg levels of lower principal quantum numbers reveal resolved multiplet structures, attributed to different fine structure components, with decreasing splitting as the ionization limit is approached. A single-Gaussian fit was applied to each resolved peak and for each unresolved multiplet. The transition energies (ν n ) of each main peak are plotted against their principal quantum number n as shown in the Fig. 3b . These data are sufficient for precise determination of the ionization limit E ′′ lim. =IP(At)− E ′′ for this excited state using the Rydberg formula: , where ν n is the transition energy from the excited state E ′′ to a Rydberg level with principal quantum number n of the valence electron, δ is the quantum defect and R M is the reduced-mass Rydberg constant for 205 At. Following the trends of quantum defects of nd and ns series of bromine and iodine [23] , we constrain the integer part to 5 or 3 for ns or nd in At, respectively. The assumption of an nd series allows us to assign principal quantum numbers to the Rydberg levels. However, the result of the analysis is unaffected by this choice. The obtained peak positions were fitted with the two free parameters E ′′ lim. and δ . The result of the fit is shown as the solid curve in the top panel of Fig. 3b . Residuals with error bars accounting for the statistical error from the Gaussian fit of each resonance and the uncertainties of the wavelength measurements are shown in the bottom panel of Fig. 3b . This approach yields E ′′ lim. =16,345.4(2) cm −1 and δ =3.16. The sum E ′′+ E ′′ lim gives the first IP of At as IP Ryd. (At)=75,150.8(7) cm −1 , corresponding to 9.31751(8) eV. Uncertainties arise from the statistical errors of 0.03 cm −1 from the Rydberg series fit and 0.09 cm −1 for the determination of E ′′. The systematic error, covering the wavelength measurements, unresolved hyperfine structure and data acquisition, is estimated to 0.6 cm −1 . This result is in perfect agreement with the preparatory direct threshold measurement but is two orders of magnitude more precise. Ab initio calculations Early predictions [10] , [11] , [12] , [13] of the IP of At at 9.2–10.4 eV were based on known IPs of other neighbouring elements and on spectroscopic data of other halogens. A compilation of all predictions involving recent calculations [14] , [15] , as well as theoretical and experimental values obtained within this work, is given in Table 1 . To strengthen this work, the IP was calculated before the experiment with the use of two relativistic methods, the multi-configuration Dirac-Fock (MCDF) and the Dirac-Coulomb (DC) coupled-cluster approach. The MCDF method provides a conceptually simple approach for computing excitation energies and IPs of heavy elements that can be improved systematically and is applicable to quite different shell structures of the atoms and ions. Although this method profits from a systematic enlargement of the active configuration space, (deep) core-valence and core-core correlations are usually not taken into account. Therefore, in recent calculations by Chang et al . [15] , the (predicted) IP was semiempirically up-shifted by 0.3 to 9.35 eV, based on similar computations for the homologue elements and the comparison with known IPs from experiment. In a more systematic treatment, we now took into account all triple excitations within the {6 s ,6 p ,6 d ,7 s ,7 p } active space as well as all single and double excitations to the { ns , np , nd , nf , ng ; n =7,8,9} orbitals, starting from the 6 s 2 6 p 5 and 6 s 2 6 p 4 reference configurations for neutral and singly charged At, respectively. In addition, core-polarization contributions from the n =4 and n =5 (fully) occupied shells were also incorporated. The most precise value obtained using this method was IP(At)=9.24(15) eV (see Table 1 ), in reasonable agreement with previous estimates. The uncertainty quoted indicates that still further correlations are expected to contribute to the IP. An alternative approach was based on the solution of the DC Hamiltonian [24] in combination with the coupled-cluster approach with single, double and perturbative triple excitations (CCSD(T)) for treatment of electron correlation. The IP was obtained by taking the energy difference between the calculated energies of the neutral element and its cation. The Dirac08 program package [25] was used to perform the calculations. The uncontracted Faegri basis sets [26] were used for At as well as for iodine (I) as a homologue, consisting of 26 s 24 p 18 d 14 f 7 g 4 h 2 i orbitals for I and 28 s 26 p 20 d 15 f 7 g 4 h 2 i orbitals for At. The convergence of the calculated IPs with respect to the size of the basis set was verified. The outer 38 electrons of I and 54 electrons of At were correlated; virtual atomic orbitals with energies higher than 50 Hartree (≈1,360 eV) were discarded. The contribution of the Breit term was assessed by performing Fock-space coupled-cluster calculations, and was found to be small: 19 cm −1 for I and 5 cm −1 for At. Higher order QED effects should thus be negligible. The final IPs, corrected for the Breit contribution, are 84,095 cm −1 for I and 75,069 cm −1 for At, corresponding to 9.307 eV. The IP value for I closely matches the experimental one of 84,295 cm −1 (refs. 23 ), and similar agreement is shown between the newly measured and CCSD(T) values for At. We apply the technique of in-source laser spectroscopy to artificially produced At isotopes. The discovered series of high-lying Rydberg states enables us to deduce the IP with high accuracy. This first experimental value of the binding energy of the valence electron of At serves as a benchmark for the prediction of the chemical properties of At as well as for predictions of atomic physics properties of the superheavy elements. The newly available, efficient three-step laser ionization scheme for At enables further experiments on At isotopes at ISOL facilities world-wide. High-resolution in-source laser spectroscopy of isotope shifts and hyperfine structures [27] as well as an extension of the study of β-delayed fission [28] to the At isotopes is in preparation. Two theoretical methods are applied to calculate the IP(At). The higher accuracy of the CCSD(T) result, compared with the MCDF value is due to better treatment of dynamic correlation within the former approach. The CCSD(T) approach is particularly suitable in this case, as the ground states of both At and At + may be approximated by single determinants. The dynamic correlation, which is handled better by CCSD(T), is the dominant effect. In-source laser spectroscopy Astatine isotopes were produced at the CERN ISOLDE radioactive ion beam facility (see ref. 20 ) by directing a 1.4-GeV pulsed proton beam of up to 2 μA from the CERN proton synchrotron booster (PSB) onto a thick target of uranium carbide (UC x ) or thorium dioxide (ThO 2 ). 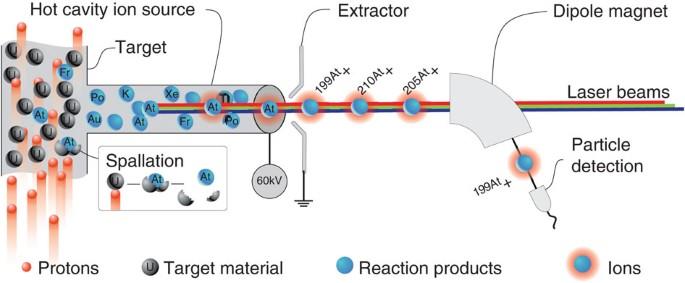Figure 4: In-source laser spectroscopy at ISOLDE. Protons impinge on a thick target inducing nuclear reactions (for example, spallation) in which different isotopes of various chemical elements are produced. The reaction products diffuse and effuse towards the hot cavity ion source, into which the precisely tuned laser beams are focussed. Step-wise resonance laser ionization creates singly charged ions of the desired element. These photo-ions are extracted and accelerated by applying a high-voltage potential. The ion beam of the isotope of interest is selected by dipole magnets and guided to a suitable detection setup. Figure 4 illustrates the in-source laser spectroscopy method. The products of the proton-induced nuclear reactions diffuse into a hot (≈2,000 °C) metal tubular cavity within which the neutral atoms are selectively photo-ionized by spatially overlapped beams of the RILIS lasers, wavelength tuned to the corresponding transitions of a photoionization scheme. Ions are extracted and accelerated by an electrostatic potential of up to 60 kV. The isotope of interest is selected by the ISOLDE mass separator dipole magnets and transmitted to the detection setups. The photo-ion signal is recorded as a function of laser frequency. Figure 4: In-source laser spectroscopy at ISOLDE. Protons impinge on a thick target inducing nuclear reactions (for example, spallation) in which different isotopes of various chemical elements are produced. The reaction products diffuse and effuse towards the hot cavity ion source, into which the precisely tuned laser beams are focussed. Step-wise resonance laser ionization creates singly charged ions of the desired element. These photo-ions are extracted and accelerated by applying a high-voltage potential. The ion beam of the isotope of interest is selected by dipole magnets and guided to a suitable detection setup. Full size image RILIS laser setup The RILIS laser system comprises tunable nanosecond dye (type Sirah Credo) and Ti:Sa lasers, pumped by the second harmonic output of Nd:YAG lasers at a pulse repetition rate of 10 kHz. The wavelengths required for excitation and ionization of the atoms were provided by the fundamental output of the lasers or by the generation of their higher harmonics. A detailed description of the RILIS laser system can be found in Fedosseev et al . [29] , Rothe et al . [30] and references therein. Spectroscopy using the Windmill detector For the initial laser spectroscopy using the inefficient two-colour scheme (cf. Fig. 1a ), a sensitive α-decay spectroscopy setup (Windmill detector), as described in Andreyev et al . [28] , was used to detect photo-ion rates in the range of 0.1–1,000 s −1 . The Windmill detector was installed at the end point of one of the beam-lines of the ISOLDE general purpose separator. The ion beam was implanted into one of ten carbon foils (20 μg cm −2 ), which are mounted on a rotating wheel. The carbon foil is surrounded by two Si-detectors to acquire the α-decay spectrum of the implanted sample. The isotope 199 At was chosen for its suitable half-life of 7.2 s and a well-separated α-decay energy of 6,643 keV. The number of 6,634 keV α-decays was counted for every wavelength combination of the RILIS dye lasers. This measurement sequence was synchronized to the PSB supercycle (≈60 s), ensuring steady conditions. Rydberg spectroscopy using FC detection For the laser spectroscopy of Rydberg states, the Ti:Sa lasers were used to generate wavelengths required for the first and second-step transition. The laser powers measured on the laser table were 33 mW (fourth harmonic) for the first step and 2 W (fundamental) for the second-step transition. The dye laser (Sirah Credo with DCM dye dissolved in ethanol) was scanned in the range of 16,599–15,523 cm −1 in two sections at a speed of −0.251 cm −1 s −1 and −0.132 cm −1 s −1 . The laser wavelengths were continuously measured with a wavelength metre (HighFinesse-Ångstrom WS/7), calibrated with a frequency stabilized HeNe laser. The three-colour ionization scheme has a higher efficiency and the photo-ion signal was obtained from a direct ion current measurement with a FC installed in the focal plane of the separator magnet. The best signal to noise ratio was obtained with the separator magnet set to transmit mass A =205. This is because of the relatively high production cross section of the isotope 205 At, its slow component of release from the ISOLDE target and relatively long half-life (26.2 min), which ensures quasi-independence from the PSB supercycle sequence. The continuous scanning method requires a correction for the integration time of the FC and potential delays in the data acquisition. The correction factor was determined separately by spectroscopy of stable manganese isotopes under the same conditions. How to cite this article: Rothe, S. et al . Measurement of the first ionization potential of astatine by laser ionization spectroscopy. Nat. Commun. 4:1835 doi: 10.1038/ncomms2819 (2013).